MLL1 is required for PAX7 expression and satellite cell self-renewal in mice PAX7 is a paired-homeobox transcription factor that specifies the myogenic identity of muscle stem cells and acts as a nodal factor by stimulating proliferation while inhibiting differentiation. We previously found that PAX7 recruits the H3K4 methyltransferases MLL1/2 to epigenetically activate target genes. Here we report that in the absence of Mll1 , myoblasts exhibit reduced H3K4me3 at both Pax7 and Myf5 promoters and reduced Pax7 and Myf5 expression. Mll1 -deficient myoblasts fail to proliferate but retain their differentiation potential, while deletion of Mll2 had no discernable effect. Re-expression of PAX7 in committed Mll1 cKO myoblasts restored H3K4me3 enrichment at the Myf5 promoter and Myf5 expression. Deletion of Mll1 in satellite cells reduced satellite cell proliferation and self-renewal, and significantly impaired skeletal muscle regeneration. Pax7 expression was unaffected in quiescent satellite cells but was markedly downregulated following satellite cell activation. Therefore, MLL1 is required for PAX7 expression and satellite cell function in vivo. Furthermore, PAX7, but not MLL1, is required for Myf5 transcriptional activation in committed myoblasts. Skeletal muscle has a remarkable capacity of regeneration that relies on a population of muscle stem cells termed satellite cells [1] . In resting adult muscle, satellite cells are mainly quiescent, but are poised for activation, allowing for muscle repair upon injury [2] . Activated satellite stem cells undergo asymmetric cell divisions to generate myogenic progenitor cells that proliferate and eventually differentiate by either fusing into damaged myofibers or generating new myofibers [3] . In addition, a subset of activated satellite cells will withdraw from the cell cycle and return to quiescence to replenish the muscle stem cell reservoir. Satellite cell function is highly regulated by extrinsic growth factors from the muscle stem cell niche as well as intrinsic transcriptional factors such as the paired-homeobox transcription factor PAX7 and the myogenic regulatory factors (MRFs) [4] . PAX7 is expressed by all satellite cells and is required for satellite cell function. Pax7 −/− mice exhibit smaller myofibers at birth and fail to form a functional muscle stem cell reservoir, leading to impaired muscle regeneration and juvenile mortality [5] , [6] , [7] , [8] . Furthermore, conditional Pax7 deletion in adult mice strongly impairs the regenerative capacity of skeletal muscle due to proliferation defects and precocious differentiation of satellite cells, confirming the absolute requirement of PAX7 for satellite cell function [9] , [10] . Chromatin immunoprecipitation (ChIP)-sequencing in primary myoblasts revealed that PAX7 acts as a nodal factor by activating target genes involved in establishing myogenic identity and in stimulating proliferation while inhibiting differentiation [11] , [12] . A major target gene of PAX7 is Myf5 , and loss of PAX7 significantly decreases Myf5 expression in both satellite cells and cultured myoblasts [6] , [9] , [11] , [13] . We previously showed that Myf5 transcriptional regulation by PAX7 involves the recruitment of the Trithorax complex, encompassing ASH2L, WDR5, RBBP5, and MLL1/2, to Myf5 regulatory sequences through direct interaction between PAX7 and MLL1/2 [13] , [14] . MLL1/2 are closely related members of a family of six histone methyltransferases that specifically methylate histone H3 lysine 4 to an activating trimethyl state (H3K4me3) [15] , [16] . The ability of PAX7 to recruit this Trithorax complex to chromatin is regulated by CARM1 and p38γ MAPK [14] , [17] . Consistent with these findings, the Myf5 locus exhibits H3K4me3 enrichment around the transcription start site (TSS) in quiescent satellite cells as well as in primary myoblasts [12] , [13] , [18] . In this study, we uncover a specific role of MLL1 in regulating PAX7 expression, elucidating their involvement in Myf5 transcriptional control. Using conditional alleles of Mll1 and Mll2 , we find that MLL1 directly regulates Pax7 . In the absence of Mll1 , myoblasts display reduced H3K4me3 enrichment at both Pax7 and Myf5 loci associated with the loss of Pax7 and Myf5 expression. As a consequence, Mll1 -deficient myoblasts fail to proliferate but retain their potential to differentiate. By contrast, deletion of Mll2 has no apparent effect. Re-establishing PAX7 expression in committed Mll1 cKO myoblasts is sufficient to restore H3K4me3 enrichment at the Myf5 promoter and rescue Myf5 levels, indicating that PAX7, but not MLL1, is required for Myf5 expression in committed myoblasts. Finally, conditional Mll1 deletion in satellite cells dramatically impairs satellite cell proliferation, self-renewal, and skeletal muscle regeneration. Altogether, our data demonstrate that MLL1 is absolutely required for PAX7 expression and satellite cell function. Loss of MLL1 impairs Pax7 and Myf5 expression Both MLL1 ( Kmt2a ) and MLL2 ( Kmt2b ) can interact with PAX7 to activate Myf5 expression [13] , [14] , suggesting that MLL1 and MLL2 may be functionally redundant. Thus, we investigated whether MLL1 and MLL2 share the same function in regulating Myf5 expression using Mll1 and Mll2 conditional knockout myoblasts ( Mll1 cKO and Mll2 cKO) and Mll1:Mll2 double conditional knockout myoblasts ( Mll1:Mll2 dcKO), derived from Rosa CE/+ :Mll1 fl/fl , Rosa CE/+ :Mll2 fl/fl and Rosa CE/+ :Mll1 fl/fl :Mll2 fl/fl mice respectively. Myoblasts were treated for 7 days with 4-hydroxytamoxifen (4OHT) followed by a 2-day washout period (Supplementary Fig. 1a ). The efficiency of Mll1 and Mll2 deletion was assessed at the RNA level (Fig. 1a–c ), and the loss of MLL1 was further confirmed at the protein level (Supplementary Fig. 1b, c ). Fig. 1 MLL1 is required for Myf5 and Pax7 expression in primary myoblasts. a – c Relative expression of Mll1 , Mll2 , Myf5 , and Pax7 in a Mll1 cKO, b Mll2 cKO, and c Mll1:Mll2 dcKO primary myoblasts and their respective controls, as determined by RT-qPCR. Data are presented as the mean ± S.E.M. of four independent experiments. d Microarray analysis was performed on control and Mll1 cKO primary myoblasts. A total of 35,557 probes were identified in the samples and plotted. e Relative expression of Myod1 , myogenin , as well as PAX7 and MLL1 target genes in control and Mll1 cKO primary myoblasts, as determined by RT-qPCR. Data are presented as the mean ± S.E.M. of four independent experiments Full size image RT-qPCR analysis revealed that Myf5 mRNA was strikingly decreased in Mll1 cKO and Mll1:Mll2 dcKO myoblasts while its expression remained unchanged in Mll2 cKO myoblasts, indicating that MLL1, but not MLL2, regulates Myf5 expression in primary myoblasts (Fig. 1a–c ). Interestingly, we also observed a mild but significant decrease of Pax7 mRNA level in both Mll1 cKO and Mll1:Mll2 dcKO myoblasts (Fig. 1a, c ), indicating that MLL1 may also regulate Pax7 transcription. As we previously demonstrated that Myf5 is a target gene of the PAX7 transcription factor [11] , [13] , our current results could suggest that Myf5 downregulation is due to a decrease in Pax7 expression. To broadly examine changes in gene expression occurring after Mll1 deletion in primary myoblasts, we used microarray to compare RNA expression in control and Mll1 cKO myoblasts obtained after a 7-day culture period with either vehicle or 4-hydroxytamoxifen, respectively (Fig. 1d , Supplementary Fig. 1d ). 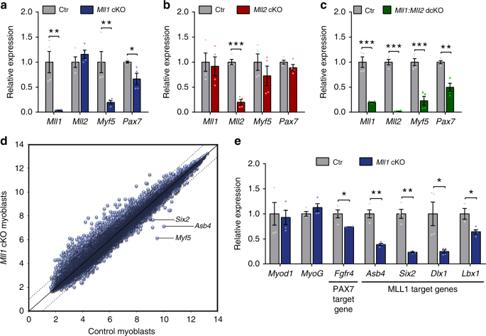Fig. 1 MLL1 is required forMyf5andPax7expression in primary myoblasts.a–cRelative expression ofMll1,Mll2,Myf5, andPax7inaMll1cKO,bMll2cKO, andcMll1:Mll2dcKO primary myoblasts and their respective controls, as determined by RT-qPCR. Data are presented as the mean ± S.E.M. of four independent experiments.dMicroarray analysis was performed on control andMll1cKO primary myoblasts. A total of 35,557 probes were identified in the samples and plotted.eRelative expression ofMyod1,myogenin, as well as PAX7 and MLL1 target genes in control andMll1cKO primary myoblasts, as determined by RT-qPCR. Data are presented as the mean ± S.E.M. of four independent experiments In Mll1 cKO myoblasts, 281 genes (322 probe sets) had a greater than twofold increase in expression, while 26 genes (29 probe sets), of which only 21 were for protein coding mRNAs, showed a greater than twofold decrease in gene expression (Table 1 ; Supplementary Data 1 ). Microarray confirmed that Pax7 expression was decreased in Mll1 cKO myoblasts (Table 1 ). Remarkably, among all the probe sets, Myf5 mRNA level displayed the greatest decrease (more than 10-fold). Initiation of myogenic differentiation coincides with both Pax7 and Myf5 downregulation, and myogenin upregulation [19] . However, myogenin mRNA level was unchanged in Mll1 cKO myoblasts (Fig. 1e ; Table 1 ), ruling out the possibility that loss of MLL1 leads to precocious myogenic differentiation. Little to no change was observed in the expression of other genes involved in myogenesis, including Myod1 (Fig. 1d, e ; Table 1 ). Interestingly, among the downregulated genes, 43% (9 out of 21) were direct MLL1 target genes in myoblasts [20] , 4 of which were also Pax7 target genes [11] . RT-qPCR in Mll1 cKO myoblasts further confirmed the downregulation of several MLL1 target genes ( Asb4 , Six2 , Dlx1 and Lbx1 ) as well as MLL1 and PAX7 common target genes ( Fgfr4 and Myf5 ) [11] , [20] , [21] (Fig. 1e ; Table 1 ). Table 1 Partial list of genes differentially expressed in Mll1 cKO and control primary myoblasts Full size table Together, our data suggest that MLL1, but not MLL2, regulates Pax7 transcription in primary myoblasts. The reduced Pax7 expression in Mll1 -deficient myoblasts could also explain the decreased expression of its target genes, Myf5 and Fgfr4 . MLL1 binds both Pax7 and Myf5 genomic loci MLL1 possesses a specific methyltransferase activity responsible for the deposition of an active tri-methylation mark on the histone H3 lysine 4 (H3K4me3) allowing for the transcriptional activation of its target genes [22] . In primary myoblasts, MLL1 bound Pax7 and Myf5 loci near the transcriptional start site (Supplementary Fig. 2a ). MLL1 also bound Pax7 +11.5 and +11.7 kb regions, which were previously shown to display H3K4me3 marks [23] . This result suggests that MLL1 can methylate the chromatin over both Pax7 and Myf5 promoters. To determine whether MLL1 binding corresponds to H3K4me3 enrichment at both Myf5 and Pax7 loci, we performed chromatin immunoprecipitation (ChIP)-qPCR using an anti-H3K4me3 antibody in control and Mll1 cKO myoblasts, and analyzed H3K4me3 enrichment at Pax7 and Myf5 promoters (Fig. 2a, b ). Mll1 deletion resulted in a clear and extensive decrease in H3K4me3 marks at the Myf5 locus (Fig. 2c ). A modest decrease in H3K4me3 enrichment was also observed at the Pax7 locus (Fig. 2c ), consistent with our RT-qPCR data showing a moderate decrease in Pax7 mRNA level. More generally, we analyzed the total level of the histone H3 and the H3K4me3 mark between control and Mll1 cKO myoblasts (Supplementary Fig. 2 b–d). H3K4me3 immunoblot analysis did not reveal any differences (Supplementary Fig. 2d ), suggesting that the loss of H3K4me3 following Mll1 deletion is gene-specific rather than global in primary myoblasts. This was expected since there was only a small number of genes downregulated upon Mll1 deletion (Table 1 , Supplementary Data 1 ). Fig. 2 Loss of MLL1 decreases H3K4me3 marks at Myf5 and Pax7 loci in Mll1 cKO myoblasts. a Location of primer sets relative to Myf5 transcription start site (TSS) for ChIP-qPCR analysis of Myf5 promoter. b Location of primer sets relative to Pax7 TSS and its downstream region for ChIP-qPCR analysis of Pax7 promoter. c ChIP-qPCR analysis of H3K4me3 enrichment, normalized to total H3, at Myf5 and Pax7 loci in control and Mll1 cKO myoblasts, obtained after 4OHT-treated or EtOH-treated Rosa CE/+ :Mll1 fl/fl myoblasts ( n = 5 independent experiments). IgH enhancer region is used as a negative control. Percent change in H3K4me3 enrichment between control and Mll1 cKO myoblasts is indicated for each region Full size image Loss of MLL1 strongly impairs myoblast proliferation Our gene expression analysis revealed that Mll1 deletion leads to a 40% decrease in Pax7 mRNA expression. Interestingly, while 90% of the control myoblasts expressed PAX7 by immunostaining, only 30% of Mll1 cKO myoblasts displayed a detectable signal for PAX7 (Fig. 3a, b ; Supplementary Fig. 3a, b ). Accordingly, western blot analysis revealed that PAX7 protein level was dramatically decreased in Mll1 cKO myoblasts as compared with control (Fig. 3c, d ). Since loss of the PAX7 transcription factor results in reduced proliferation [9] , we assessed the proliferation of Mll1 cKO myoblasts. After 6 days of culture, Mll1 cKO myoblasts underwent a modest 3.5-fold expansion while control myoblasts expanded by 40-fold (Fig. 3e ). To further confirm the impairment of proliferation following Mll1 deletion, myoblasts were immunostained with the cell proliferation marker Ki67 (Fig. 3a ). Mll1 cKO myoblasts showed a twofold decrease in the proportion of Ki67-positive cells compared with the control (Fig. 3f ). Fig. 3 Loss of MLL1 abolishes PAX7 expression and myoblast proliferation, but does not affect myogenic differentiation. a Immunostaining of PAX7 (green) and Ki67 (red) in control and Mll1 cKO primary myoblasts. Nuclei are counterstained with DAPI (blue). Scale bars represent 20 µm. b Quantification of PAX7-expressing cells from control and Mll1 cKO primary myoblasts. Data are presented as the mean ± S.E.M. of three independent experiments. c Western blot analysis of PAX7 and MYOD in control and Mll1 cKO primary myoblasts. GAPDH is used as a loading control. d Densitometric analysis of the relative levels of PAX7 normalized to GAPDH signals of six independent experiments. Values are represented as the mean ± S.E.M. e Control and Mll1 cKO primary myoblasts were plated at the same density and grown for 6 days. Every 2 days, cells were numerated to evaluate their proliferation, represented as the mean ( n = 3 biological replicates) ± S.E.M. f Quantification of Ki67-expressing cells from control and Mll1 cKO primary myoblasts. Data are presented as the mean ( n = 3 biological replicates) ± S.E.M. g Western blot analysis of Myosin Heavy Chains (MHC) and MYOGENIN during differentiation of control and Mll1 cKO primary myoblasts. TUBULIN is used as a loading control. h Immunostaining of MHC (green) and PAX7 (red) in control and Mll1 cKO primary myoblasts cultured in differentiation medium for 6 days. Nuclei are counterstained with DAPI (blue). Scale bar represents 100 µm Full size image We also evaluated the capacity of Mll1 cKO myoblasts to differentiate. Either MYF5 or MYOD are capable of activating the myogenic program [24] . Although Mll1 deletion resulted in loss of Myf5 expression, Mll1 cKO myoblasts still expressed MYOD as well as other myogenic markers such as SYNDECAN-4 (SDC4) (Fig. 3c ; Table 1 ; Supplementary Fig. 3a, b ). This result indicates that Mll1 cKO myoblasts retained myogenic competence. Mll1 cKO myoblasts plated at high confluency were able to differentiate, expressing both MYOGENIN and myosin heavy chain (MHC) (Fig. 3g ; Supplementary Fig. 3c ), and to fuse normally into myotubes (Fig. 3h ). Nevertheless, after 6 days of differentiation, a pool of PAX7-expressing mononucleated myoblasts, or reserve cells, arose alongside the control myotubes whereas it was absent after Mll1 deletion (Fig. 3h ). Taken together, this suggests that MLL1 is required to generate the reserve progeny upon differentiation. These results demonstrate that MLL1 is required for PAX7 expression and proliferation of myogenic progenitor cells, but is dispensable for differentiation. Exogenous Pax7 rescues Myf5 expression in Mll1 cKO myoblasts Mll1 cKO myoblasts display more than 10-fold lower levels of Myf5 transcript than control myoblasts and scarcely express Pax7 protein (Figs. 1 and 3 ). The PAX7 transcription factor is known to recruit the Trithorax complex to Myf5 regulatory sequences through a direct interaction with MLL1/2 [13] , [14] . As PAX7 is required for Myf5 expression [11] , [13] , we hypothesized that the decrease of Myf5 transcription in Mll1 cKO primary myoblasts is directly attributed to the loss of PAX7 rather than the loss of MLL1. Hence, we asked whether the downregulation of Myf5 expression in Mll1 cKO myoblasts could be rescued by PAX7 overexpression solely. To address this question, we generated stable Rosa CE/+ :Mll1 fl/fl cell lines overexpressing either an empty plasmid (CMV-empty) or Pax7 (CMV-Pax7), and we subsequently treated these lines with either vehicle (control) or 4-hydroxytamoxifen ( Mll1 cKO) (Supplementary Fig. 4a ). Mll1 deletion was confirmed at both RNA and protein levels (Supplementary Fig. 4 b–d). As expected, upon 4-hydroxytamoxifen treatment, Rosa CE/+ :Mll1 fl/fl cells expressing the empty plasmid exhibited a 40% decrease and a 90% decrease in Pax7 and Myf5 transcripts, respectively (Fig. 4b, c ). Consistent with our previous finding, PAX7 protein was barely detectable (Fig. 4a ; Supplementary Fig. 4c ). Compared with the control lines, CMV-Pax7 transduced myoblasts had increased and stable PAX7 expression at both RNA and protein levels independently of Mll1 deletion (Fig. 4a, b ; Supplementary Fig. 4c ). Pax7 -overexpressing myoblasts also exhibited increased Myf5 expression compared with the myoblasts transduced with the empty vector (Fig. 4c ). Importantly, deletion of Mll1 in Pax7 -overexpressing myoblasts neither changed Myf5 expression, nor H3K4me3 enrichment at the Myf5 locus (Fig. 4c, d ), demonstrating that the loss of Myf5 expression and H3K4me3 at the Myf5 locus in Mll1 cKO myoblasts is a consequence of the absence of PAX7. Of note, Pax7 overexpression in Mll1 cKO myoblasts did not rescue the expression of the MLL1 target genes Six2 , Dlx1 , Lbx1 , or Asb4 , as their expression was decreased in Pax7 -overexpressing cells following Mll1 deletion (Fig. 4e ). However, this phenotype was not observed for the PAX7 target gene Fgfr4 [11] (Fig. 4e ). This indicates that Mll1 deletion results in changes in gene expression that can be partially rescued by PAX7, and suggests that other histone methyltransferases can compensate for the absence of MLL1 to activate PAX7 target genes in Mll1 cKO myoblasts. Fig. 4 Overexpression of PAX7 restores Myf5 expression and H3K4me3 marks at Myf5 locus in Mll1 cKO myoblasts. a Immunostaining of PAX7 (green) and Ki67 (red) in control and Mll1 cKO primary myoblasts transduced with either an empty plasmid or a CMV-Pax7 plasmid. Nuclei are counterstained with DAPI (blue). Scale bars represent 20 µm. b , c RT-qPCR analysis of ( b ) Pax7 and ( c ) Myf5 mRNA expression performed on control and Mll1 cKO primary myoblasts transduced with either an empty plasmid or a CMV-Pax7 plasmid, represented as mean ± S.E.M. ( n = 4 independent experiments). d ChIP-qPCR analysis of H3K4me3 enrichment, normalized to H3, at Myf5 locus in control and Mll1 cKO primary myoblasts transduced with either an empty plasmid or a CMV-Pax7 plasmid. Values represent mean ± S.E.M. ( n = 3 independent experiments). IgH enhancer region is used as a negative control. e Relative expression of PAX7 and MLL1 target genes in control and Mll1 cKO primary myoblasts transduced with either an empty plasmid or a CMV-Pax7 plasmid, represented as mean ± S.E.M. ( n = 4 independent experiments). f Number of control and Mll1 cKO primary myoblasts transduced with either an empty plasmid or a CMV-Pax7 plasmid. Cells were plated at the same density and grown for 6 days before enumeration. Values represent mean ± S.E.M. ( n = 4 independent experiments) Full size image In order to evaluate whether another histone methyltransferase (HMT) can substitute for MLL1 in regulating the expression of PAX7 and its target genes, we transiently transfected primary myoblasts with siRNAs targeting Mll1 alone or in combination with siRNAs targeting Mll2 , Set1a , and Set1b , which are known to mediate H3K4 tri-methylation at gene promoters [15] , [16] (Supplementary Fig. 4e, f ). As a control, we first tested the capacity of the four individual HMTs to regulate Pax7 and Myf5 transcription (Supplementary Fig. 4e ). We observed that only Mll1 knockdown leads to a decrease in both Pax7 and Myf5 expression (Supplementary Fig. 4e ), recapitulating our first observations (Fig. 1 ). Interestingly, co-transfection of Mll1 siRNA with either Mll2 siRNA or Set1b siRNA further decreased Pax7 and Myf5 expression, while the combination of Mll1 and Set1a siRNA did not show any effect compared with the treatment with Mll1 siRNA only (Supplementary Fig. 4f ). Thus, these results suggest that in Mll1 cKO myoblasts, MLL2 and SET1B can compensate and substitute for MLL1 in regulating Pax7 and Myf5 RNA levels. Consistent with the finding that PAX7 regulates myoblast proliferation [9] , Pax7 -overexpressing myoblasts exhibited increased proliferation compared with the myoblasts transduced with the empty vector (Fig. 4f ). However, the proliferation defect observed in Mll1 cKO myoblasts was only partially rescued by PAX7 overexpression as demonstrated by Ki67 immunostaining and proliferation assay (Fig. 4a, f ). Taken together, our data confirm that MLL1 is required for PAX7 expression and myoblast proliferation, and that PAX7 expression is sufficient to restore the transcription of its target genes. In contrast, the proliferation defect in Mll1 cKO myoblasts is partially rescued by PAX7 suggesting that MLL1 can mediate cell proliferation independently of PAX7. Mll1 deletion in satellite cells impairs muscle regeneration PAX7 is required for satellite cell function in adult skeletal muscle [5] , [7] , [9] , [10] . Since PAX7 expression is compromised in Mll1 cKO myoblasts, we investigated the role of MLL1 in satellite cell function in vivo. To this end, we generated Pax7 CE/+ :Mll1 fl/fl :Rosa YFP mice allowing for tamoxifen-inducible genetic deletion of Mll1 in Pax7 -expressing cells (Supplementary Fig. 5a ). Pax7 CE/+ :Mll1 fl/fl :Rosa YFP mice were intraperitoneally injected with tamoxifen for 4 consecutive days and kept on a tamoxifen diet thereafter (Fig. 5a ). Since our in vitro data revealed that MLL1 is required for both PAX7 expression and myoblast proliferation, Pax7 CE/+ :Mll1 fl/fl :Rosa YFP mice were maintained on tamoxifen diet throughout the experimental time course to prevent growth of satellite cells escaping from tamoxifen-induced Mll1 recombination [9] . Non-tamoxifen-treated Pax7 CE/+ :Mll1 fl/fl :Rosa YFP mice were used as controls. One week after the first tamoxifen injection, the efficiency of Mll1 deletion was determined by RT-qPCR on freshly isolated quiescent satellite cells and activated satellite cells sorted 3 days after cardiotoxin (CTX)-induced injury (Supplementary Fig. 5b, d ). Although Mll1 was significantly downregulated in quiescent satellite cells after tamoxifen treatment, we did not observe differences in the expression of Pax7 and its target genes Myf5 and Fgfr4 , while the expression of MLL1 target genes were downregulated (Supplementary Fig. 5b ). Moreover, H3K4me3 enrichment was unchanged at both Pax7 and Myf5 loci (Supplementary Fig. 5c ). Together, these results suggest that MLL1 does not regulate PAX7 expression in quiescent satellite cells. Fig. 5 Genetic deletion of Mll1 in satellite cells strongly impairs muscle regeneration. a Experimental schematic outlining the protocol followed to analyzed muscle regeneration of Pax7 CE/+ :Mll1 fl/fl mice. b Hematoxylin and eosin (H&E) staining of cardiotoxin (CTX)-injured and contralateral (ctr) tibialis anterior (TA) muscles from Pax7 CE/+ :Mll1 fl/fl mice, treated or not with tamoxifen at 7 days or 21 days post-injury. Scale bar represents 100 µm. c Wheat germ agglutinin (WGA, red) and DYSTROPHIN (green) staining of CTX-injured and contralateral TA muscles from Pax7 CE/+ :Mll1 fl/fl mice, treated or not with tamoxifen at 7 days or 21 days post-injury. Nuclei are stained with DAPI (blue). Scale bar represents 100 µm. d Relative CTX-injured and contralateral (ctr) TA muscle weight normalized to the body weight at 21 days post-injury, represented as means ± S.E.M ( n = 7 mice per group). e Myofiber minimal Feret’s diameter of CTX-injured and contralateral (ctr) TA muscles from Pax7 CE/+ :Mll1 fl/fl mice treated or not with tamoxifen at 21 days post-injury, represented as mean ± S.E.M ( n = 7 mice per group). f Distribution of minimal Feret’s diameter of CTX-injured TA muscles, as determined in e Full size image However, as observed for the Mll1 cKO primary myoblasts, RT-qPCR revealed that the expression of Pax7 and its target genes Myf5 and Fgfr4 was significantly downregulated in Mll1 -deficient activated satellite cells (Supplementary Fig. 5d ). MLL1 target genes were also downregulated. Consistent with the RT-qPCR data, H3K4me3 enrichment was decreased at both Pax7 and Myf5 loci in activated satellite cells (Supplementary Fig. 5e ). Together, these data indicate that MLL1 is important in regulating Pax7 expression upon satellite cell activation. We also addressed whether Mll1 deletion impairs satellite cell function by studying the capacity of Mll1 cKO satellite cells to regenerate the muscle after an injury. Muscle regeneration was assessed at 7 days and 21 days following acute injury induced by cardiotoxin (CTX) injection into the tibialis anterior (TA) muscle (Fig. 5a ). Hematoxylin and eosin (H&E) and wheat germ agglutinin (WGA) staining on muscle cross-sections revealed evident histological differences in tamoxifen-treated Pax7 CE/+ :Mll1 fl/fl :Rosa YFP mice associated with increased fibrotic deposits at 7 days post-injury (d.p.i.) and smaller myofibers at 21 d.p.i. (Fig. 5b, c ). Tamoxifen-treated Pax7 CE/+ :Mll1 fl/fl :Rosa YFP mice exhibited a 30% decrease in injured muscle weight compared with the control mice at 21 d.p.i. (Fig. 5d ; Supplementary Fig. 5f ). While the total number of myofibers in injured muscles was unchanged (Supplementary Fig. 5g ), myofiber minimal Feret’s diameter was significantly decreased in tamoxifen-treated mice at 21 d.p.i. (Fig. 5e, f ). No differences were observed in the uninjured contralateral muscles, consistent with the hypothesis that MLL1 does not regulate PAX7 in the quiescent stem cell pool. Taken together, our results indicate that loss of MLL1 in satellite cells strongly impairs muscle regeneration. MLL1 is required for satellite cell self-renewal The impairment in muscle regeneration implies defects in satellite cell function of tamoxifen-treated Pax7 CE/+ :Mll1 fl/fl :Rosa YFP mice. Therefore, we analyzed the functional consequences of Mll1 deletion in satellite cells. At 7 d.p.i., we enumerated the numbers of proliferating and differentiating satellite cells expressing either PAX7 or MYOGENIN (MYOG), respectively (Fig. 6a ). Enumeration of PAX7-positive cells revealed a dramatic fourfold decrease in satellite cell numbers (Fig. 6b ), consistent with reduced cell proliferation. At 7 d.p.i., tamoxifen-treated Pax7 CE/+ :Mll1 fl/fl :Rosa YFP mice also exhibited a twofold decrease in the numbers of MYOGENIN-expressing cells (Fig. 6c ). The loss of MYOG-expressing cells could be a consequence of the reduced number of satellite cells. Alternatively, it could suggest a differentiation defect of Mll1 -deficient satellite cells. At the end of the regeneration process at 21 d.p.i., the number of PAX7-expressing satellite cells was reduced by sixfold in tamoxifen-treated Pax7 CE/+ :Mll1 fl/fl :Rosa YFP mice (Fig. 6d, e ), suggesting that Mll1 knockout satellite cells failed to self-renew and Mll1 deletion led to the loss of the satellite stem cell pool. Fig. 6 MLL1 is required for satellite cell proliferation and maintenance of the satellite cell pool. a Immunostaining with PAX7 (red) and MYOGENIN (orange) showing a markedly reduced numbers of satellite cells (white arrows) and differentiated cells (empty arrows) after satellite cell-specific deletion of Mll1 induced by tamoxifen treatment. DYSTROPHIN staining (green) delineates the myofibers. Nuclei are counterstained with DAPI (blue). Scale bar represents 50 µm. b Quantification of Pax7-expressing cells per mm² from injured TA muscles of untreated ( n = 6 mice) or tamoxifen-treated ( n = 5 mice) Pax7 CE/+ :Mll1 fl/fl mice at 7 days post-injury. c Quantification of MYOGENIN-expressing cells per mm² from injured TA muscle sections of untreated ( n = 6 mice) or tamoxifen-treated ( n = 5 mice) Pax7 CE/+ :Mll1 fl/fl mice 7 days post-injury. d Immunostaining with PAX7 (red) confirming the decreased number of satellite cells (white arrows) after satellite cell-specific deletion of Mll1 induced by tamoxifen treatment. DYSTROPHIN staining (green) delineates the myofibers. Nuclei are counterstained with DAPI (blue). Scale bar represents 50 µm. e Quantification of Pax7-expressing cells per mm² from injured TA muscle sections of untreated or tamoxifen-treated Pax7 CE/+ :Mll1 fl/fl mice 21 days post-injury ( n = 4 mice per group) Full size image To examine the fate of satellite cells in tamoxifen-treated Pax7 CE/+ :Mll1 fl/fl :Rosa YFP mice during muscle regeneration, we took advantage of the Rosa YFP allele to label PAX7-expressing Mll1 -deficient satellite cells and trace them during muscle regeneration (Supplementary Fig. 5a ). One week after the first tamoxifen injection, immunostaining on muscle cross-sections revealed that YFP was expressed specifically in PAX7-expressing satellite cells in tamoxifen-treated Pax7 CE/+ :Mll1 fl/fl :Rosa YFP mice (Fig. 7a ; Supplementary Fig. 6a ). No YFP expression was detected in non-tamoxifen-treated mice. At 7 d.p.i., YFP-positive cells adjacent to the regenerating myofibers were detected, all of them expressing either PAX7 or MYOG (Fig. 7b ). Interestingly, YFP was also expressed in the majority of regenerating myofibers marked by the expression of the embryonic MHC (eMHC) (Fig. 7b ; Supplementary Fig. 6b ), suggesting that YFP-positive satellite cells were able to differentiate. At 21 d.p.i., the regenerated myofibers were all labeled by YFP, while only very rare YFP-positive PAX7-positive satellite cells were observed (Fig. 7c ; Supplementary Fig. 6c ). No interstitial YFP-positive cells were found. These observations demonstrate that Mll1 -deficient satellite cells successfully differentiated and fused into new myofibers while they were not able to self-renew. Interestingly, the number of PAX7-positive satellite cells co-expressing YFP in the contralateral (uninjured) muscle was unchanged from day 0 to day 21 post-injury (Supplementary Fig. 6 ) confirming that Mll1 deficiency had no effect on PAX7 expression in the quiescent satellite cell pool. Fig. 7 Mll1 -deficient satellite cells retain their capacity to differentiate during muscle regeneration. a Immunostaining of PAX7 (red) showing satellite cells co-expressing YFP (green) upon 7-day tamoxifen treatment (+Tmx) in uninjured TA muscles from Pax7 CE/+ :Mll1 fl/fl :Rosa YFP mice. Untreated mice (− Tmx) do not exhibit any YFP staining. Nuclei are stained with DAPI (blue). Scale bar represents 20 µm. b Top and mid panel: satellite cells expressing either PAX7 (red) or MYOGENIN (orange), co-stained with YFP (green), of CTX-injured TA muscles from Pax7 CE/+ :Mll1 fl/fl :Rosa YFP mice treated or not with tamoxifen at 7 days post-injury. Nuclei are counterstained with DAPI (blue). Scale bar represents 20 µm. Lower panel: immunostaining of embryonic MHC (eMHC, red) for regenerating myofibers and YFP (green) at 7 days post-injury. Scale bar represents 50 µm. c PAX7 (red) and YFP (green) immunostaining of CTX-injured TA muscles from Pax7 CE/+ :Mll1 fl/fl :Rosa YFP mice treated or not with tamoxifen at 21 days post-injury. DAPI stained the nuclei (blue). Scale bar represents 20 µm. Throughout, white arrows and empty arrows indicate wild-type and Mll1 knockout satellite cells, respectively Full size image To further confirm the loss of the satellite stem cell pool after regeneration, Pax7 CE/+ :Mll1 fl/fl :Rosa YFP mice were subjected to a second CTX injury (Supplementary Fig. 7a ). Twenty one days after the second injury, tamoxifen-treated Pax7 CE/+ :Mll1 fl/fl :Rosa YFP mice exhibited a dramatic 70% decrease in the relative muscle weight compared with the controls (Supplementary Fig. 7b, c ). The regeneration deficit was even more pronounced as evidenced by extensive fibrosis and absence of newly regenerated myofibers (Supplementary Fig. 7d–f ). Finally, no PAX7-expressing cells were found in double injured muscles while satellite cells remained present in the contralateral muscle and in animals not treated with tamoxifen (Supplementary Fig. 7g ). Therefore, these data clearly demonstrate that Mll1 deletion leads to the loss of the satellite stem cell pool after regeneration. Based on all our results, we conclude that MLL1 does not affect the quiescent stem cell pool in resting muscle. However, MLL1 is absolutely required for satellite cell proliferation and self-renewal during skeletal muscle regeneration, while it does not interfere with their capacity to differentiate. Satellite cell function relies on the transcription factor PAX7, as it regulates a large number of target genes involved in myogenic identity, growth, and proliferation [5] , [9] , [11] . In this study, we show that MLL1, but not MLL2, is absolutely required for PAX7 expression in activated satellite cells and myoblasts, but not in quiescent satellite cells. PAX7 is capable of interacting with either MLL1 or MLL2 [13] , [14] . However, only Mll1 deletion leads to a complete loss of Myf5 mRNA, while Mll2 cKO myoblasts maintain Myf5 transcription. These results indicate that in primary myoblasts, MLL2 is dispensable for Myf5 expression. Accordingly, accumulating evidence shows that the activities of MLL1 and MLL2 are restricted to selective sets of target genes in very specific cell types during development [25] , [26] , [27] . Thus, MLL2 could be considered having a role in Myf5 transcription through its interaction with PAX7 earlier during muscle development or on a distinct subset of target genes. Aside from Myf5 downregulation, our microarray analysis performed on control and Mll1 cKO myoblasts revealed remarkably little change in gene expression, even amongst Hox and homeobox genes which have been previously determined to be MLL1 targets [20] , [21] , [22] , [28] , [29] , [30] , [31] . Cultured myoblasts are committed and have limited cell-type plasticity under standard growth conditions [2] . Thus, Mll1 deletion would not result in a change in cell identity, explaining why we do not observe major modifications in Hox and homeobox gene expression. Nevertheless, we determined that 43% of the downregulated genes in Mll1 cKO myoblasts were direct MLL1 target genes [20] . In contrast, upregulation of gene expression results mostly from an indirect effect of the loss of MLL1, since only 23% (64 of 281) of the upregulated genes were bound by MLL1 in myoblasts [20] . Gene ontology analysis on the upregulated genes revealed biological process (BP) terms associated with negative regulation of biological and cellular processes such as cell proliferation or migration, as expected (Supplementary Data 2 ). It also highlighted cellular component (CC) terms associated to the myofibril, contractile fiber, and sarcomere, further confirming that Mll1 cKO cells retain myogenic identity. Our results indicate that in primary myoblasts, the absence of MLL1 leads to the downregulation of a very small subset of genes including five transcription factors ( Pax7 , Myf5 , Lbx1 , Six2 , and Dlx1 ), which in turn leads to an overall indirect increase in gene expression. Overexpression of PAX7 rescues Myf5 transcripts levels in the absence of MLL1, supporting the idea that Myf5 expression is dependent on PAX7 [11] , [13] . Moreover, PAX7 overexpression re-establishes the H3K4me3 marks on Myf5 regulatory sequences in the absence of MLL1, suggesting that some other histone methyltransferases can substitute for MLL1 in activating the Myf5 locus. Indeed, our results suggest that MLL2 and SET1B can compensate for the absence of MLL1 in regulating Myf5 expression. Several studies have highlighted the robust activity of SET1A/B methyltransferase containing complexes, which write the majority of H3K4me3 marks relative to the MLL1–4 containing complexes [32] , [33] , [34] . Therefore, SET1B may be recruited to the Myf5 promoter to activate transcription in the absence of MLL1. The mechanism by which MLL1 is recruited to the Pax7 promoter is still unknown. Chromatin immunoprecipitation experiments showed MLL1 binding to five genomic loci of the Pax7 gene (−0.2 kb, +0.6 kb, +1.1 kb, +11.5 kb, +11.7 kb). In silico analysis revealed putative binding sites for several transcription factors that are expressed in satellite cells and bind at least two different Pax7 loci, including KLF5, EWSR1, SP2, SP3, and ZFP263. Of note, an interaction between EWSR1 and MLL1 has been reported using BioID [35] , and different oncogenic fusion proteins involving EWSR1 can drive Pax7 expression in Ewing sarcomas [36] . Whether EWSR1 or other transcription factors are responsible for MLL1 recruitment to the Pax7 promoter remains to be determined. Although MLL1 binds Pax7 regulatory sequences, Mll1 deletion in primary myoblasts only results in a modest decrease of H3K4me3 at the Pax7 locus, in agreement with previous findings stating that loss of MLL1 does not always trigger H3K4me3 changes at its target genes [25] , [28] , [37] . In Mll1 cKO myoblasts, Pax7 mRNA levels are decreased by 40% compared with control, while PAX7 protein is barely detectable. Taken together, these results suggest the intriguing possibility that MLL1 contributes to PAX7 regulation through other mechanisms than its histone methyltransferase function. This hypothesis is further supported by several studies suggesting that the role of MLL1 is partly independent of its H3K4 methyltransferase activity [25] , [37] , [38] . Further studies will be required to clarify the non-HMT roles of MLL1 in muscle stem cells. In accordance with the absolute requirement for PAX7-expressing satellite cells in skeletal muscle regeneration [5] , [9] , [39] , [40] , satellite cell-specific deletion of Mll1 dramatically impaired muscle regeneration in vivo. To date, MLL1 is the first known regulator of Pax7 to display such a drastic phenotype that results in the failure in muscle regeneration and the exhaustion of the satellite stem cell pool, phenocopying the Pax7 -conditional knockout mice [9] . This appears to be largely due to a defect in satellite cell proliferation and self-renewal. Indeed, during skeletal muscle regeneration, Mll1 -deficient satellite cells fail to proliferate, but do ultimately differentiate and fuse into regenerating myofibers. At 21 days post-injury, only very rare PAX7-expressing cells were observed, which correlates with a loss of the satellite stem cell pool. This was further supported by our results following a second muscle injury that ultimately results in a profound regeneration deficit as observed in different mouse models following genetic ablation of adult muscle stem cells [39] , [40] . However, all regenerating myofibers were YFP-positive, confirming that satellite cells have differentiated at the expense of self-renewal. Together, these results confirm that MLL1 plays essential roles in the proliferation and self-renewal of satellite cells. Our data further support prior findings that MLL1 is a necessary factor for stem cell maintenance and function, and may suggest that MLL1 has important roles for other stem cell types. Previous findings show that the adult steady-state hematopoiesis relies on MLL1 activity, allowing for the maintenance of the hematopoietic stem cell (HSC) pool and promoting the proliferation of progenitors through expression of homeodomain and other transcription factors [30] , [41] . In the absence of Mll1 , HSCs exit from quiescence to precociously enter cell cycle without an increase in their number, suggesting that HSC division is accompanied by differentiation and not self-renewal [30] , [41] . Additionally, MLL1 is critical for neural development and for post-natal differentiation of neurogenic stem cells [42] , [43] . However, in contrast to HSCs and muscle stem cells, Mll1 -deficient neural stem cells are able to proliferate, but fail to activate Dlx2 to initiate the neuronal program [28] . Together, our data adds to and reinforces the understanding that MLL1 performs essential functions to regulate stem cell biology. Our work adds myogenesis to the list of stem cell dependent processes which require MLL1. Furthermore, we deciphered a new mechanism of satellite cell regulation that acts upstream of Pax7, and perturbation of this regulatory pathway leads to a profound deficit in satellite cell function. This work adds to our understanding of PAX7 transcription and the regulation of myogenesis upstream of PAX7 and may provide insight for future therapies targeting myogenic deficiencies or malignancies. Mice and animal care Mll1 fl/fl mice [30] and Mll2 fl/fl mice [44] were crossed with Rosa CE/+ mice [45] to obtain the Rosa CE/+ :Mll1 fl/fl , Rosa CE/+ :Mll2 fl/fl , and Rosa CE/+ :Mll1 fl/fl : Mll2 fl/fl mice used for the in vitro experiments. Tamoxifen-inducible Pax7 CE/+ :Mll1 fl/fl :Rosa YFP mice were generated by crossing Pax7 CE/+ mice [46] with Gt(ROSA)26Sor tm3(CAG-EYFP) (referred as Rosa YFP in the text) mice (Jackson Laboratory) and Mll1 fl/fl mice. Mice were injected intraperitoneally with 100 µL of a 20 mg.mL −1 tamoxifen solution dissolved in corn oil (Tmx, Sigma T5648) for 4 consecutive days, and maintained on tamoxifen diet (500 mg Tmx per kg diet, Teklad, Envigo). All the mice used in this study were males and females, from 6- to 16-week old, with mixed genetic background (129SV and C57BL/6). Housing, husbandry and all experimental protocols for mice used in this study were performed in accordance with the guidelines established by the University of Ottawa Animal Care Committee, which is based on the guidelines of the Canadian Council on Animal Care (CCAC). Protocols were approved by Animal Research Ethics Board (AREB) at the University of Ottawa. Muscle regeneration and histology Muscle injury was induced by injection of 50 μl of 10 µM cardiotoxin (CTX) from Naja mossambica mossambica (Latoxan, L8102) into the tibialis anterior (TA) muscle of isofluorane-anesthetized animals. For the double injury protocol, CTX was reinjected 21 days after the first injury. Seven, 21, and 42 days after CTX injections, mice were euthanized and TA muscles were harvested, weighed and embedded in OCT cooled with liquid nitrogen. For GFP visualization, mice were euthanized with a sodium pentobarbital solution (Euthanyl) and perfused with PBS before fixation with 4% paraformaldehyde (PFA) solution in PBS. Muscles were excised, further fixed into 0.1% PFA solution in PBS for 16 h, then transferred into ascending sucrose gradients (15%, 30% in PBS), and finally embedded and frozen in OCT. Embedded muscles were cryosectioned with 10 µm thickness. For fiber counting and minimal Feret’s diameter analysis, cryosections were washed with PBS, blocked in 5% goat serum, 2% BSA in PBS, stained with Wheat Germ Agglutinin Alexa647 conjugate for 1 h at room temperature and nuclei were counterstained with Hoechst (1:1000 in PBS). Images were taken on a Zeiss Axio Observer.D1 inverted microscope equipped with an EC Plan-Neofluar 10 × /0.3 Ph1 M27 objective, and stitched together using Fiji software ( http://fiji.sc/Fiji ) [47] . Stitched pictures were analyzed using the SMASH software in MATLAB 2015a [48] . Total number of myofibers in each tissue was verified manually and more than 95% of myofibers were quantified across each muscle section. Fluorescence-activated cell sorting Satellite cells were prospectively isolated by flow cytometry using Alexa647-conjugated anti-α7-Integrin, biotin-conjugated anti-CD34 (streptavidin PE-Cy7 conjugate), and PE-conjugated anti-CD31, anti-CD45, anti-SCA1, and anti-CD11b antibodies [49] . Quiescent satellite cells were obtained from uninjured hind limb muscles while activated satellite cells were obtained from CTX-injured tibialis anterior and gastrocnemius muscles 3 days after the induced injury. The list of antibodies is provided in Supplementary Table 3 . 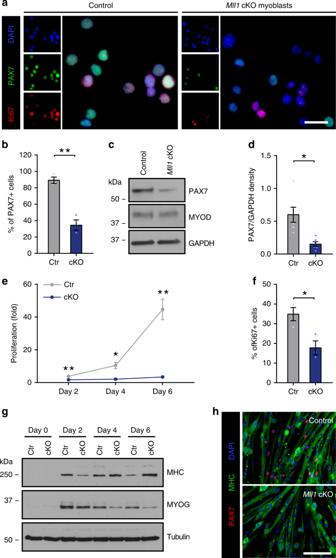Fig. 3 Loss of MLL1 abolishes PAX7 expression and myoblast proliferation, but does not affect myogenic differentiation.aImmunostaining of PAX7 (green) and Ki67 (red) in control andMll1cKO primary myoblasts. Nuclei are counterstained with DAPI (blue). Scale bars represent 20 µm.bQuantification of PAX7-expressing cells from control andMll1cKO primary myoblasts. Data are presented as the mean ± S.E.M. of three independent experiments.cWestern blot analysis of PAX7 and MYOD in control andMll1cKO primary myoblasts. GAPDH is used as a loading control.dDensitometric analysis of the relative levels of PAX7 normalized to GAPDH signals of six independent experiments. Values are represented as the mean ± S.E.M.eControl andMll1cKO primary myoblasts were plated at the same density and grown for 6 days. Every 2 days, cells were numerated to evaluate their proliferation, represented as the mean (n= 3 biological replicates) ± S.E.M.fQuantification of Ki67-expressing cells from control andMll1cKO primary myoblasts. Data are presented as the mean (n= 3 biological replicates) ± S.E.M.gWestern blot analysis of Myosin Heavy Chains (MHC) and MYOGENIN during differentiation of control andMll1cKO primary myoblasts. TUBULIN is used as a loading control.hImmunostaining of MHC (green) and PAX7 (red) in control andMll1cKO primary myoblasts cultured in differentiation medium for 6 days. Nuclei are counterstained with DAPI (blue). Scale bar represents 100 µm In brief, dissected muscles were minced in collagenase/dispase solution followed by dissociation using the gentleMACS Octo Dissociator with Heaters (Miltenyi Biotec). Cells were then filtered through a 70 µm nylon mesh and collected by centrifugation. Cell pellets were resuspended in FACS buffer (10% FBS, 5 mM EDTA in PBS) and incubated with the antibodies listed above. Unbound antibodies were washed with FACS buffer and cells were pelleted prior to resuspension in FACS buffer and a final filtration through a 30 µm filter. Satellite cells were sorted based on forward scatter and side scatter profiles, followed by negative lineage selection in PE (CD11b−, SCA1−, CD45−, CD31−) and positive selection in Alexa647 (α7-Integrin+) and PE-Cy7 (CD34+). Flow cytometry was performed using a MoFlo XDP (Beckman Coulter). The sequential gating strategy is described in Supplementary Fig. 9 . Primary myoblast isolation and culture Primary myoblasts were derived from hind limb muscles of 5–6-week-old mice by magnetic cell separation (MACS) [50] . In brief, muscle dissociation and cell filtration was performed as described above for FACS. Cell pellets were resuspended in FACS buffer and incubated with biotin-conjugated lineage antibodies (CD11b−, SCA1−, CD45−, CD31−), followed by incubation with streptavidin microbeads for negative lineage selection. Cell suspensions were loaded onto a LD column (Miltenyi Biotec) in a magnetic field of a VarioMACS separator (Miltenyi Biotec) and rinsed with FACS buffer. Column flow-through was collected and then stained with biotin-conjugated anti-α7-Integrin antibody, followed by incubation with streptavidin microbeads, to purify the satellite cell-derived myoblasts. Cells were loaded onto a MS column (Miltenyi Biotec) and washed three times with FACS buffer. Flow-through containing unlabeled cells was discarded, and the column was flushed to collect positively labeled satellite cell-derived myoblasts. Myoblasts were cultured on collagen-coated dishes in Ham’s F10 medium (Wisent, 318-051-CL) supplemented with 20% FBS, 1% penicillin/streptomycin, and 5 ng.mL −1 of basic FGF (Millipore, GF003AFMG). For in vitro knockout experiments, myoblasts were treated with 500 nM (Z)−4-Hydroxytamoxifen (4OHT, resuspended in ethanol (Sigma, H7904-5MG)), for 7 days followed by 2 days of culture in the absence of 4OHT prior to collection of cells for analysis. Differentiation was triggered in Ham’s F10:DMEM 1:1 (Wisent, 319-016-CL) supplemented with 5% horse serum, and 1% penicillin/streptomycin. Primary myoblast transfection To obtain the Pax7 -overexpressing primary myoblasts, Pax7 cDNA was cloned into the pHAN backbone (with puromycin resistance driven from a distinct SV40 promoter) [13] . Control virus expressed puromycin resistance alone. Retrovirus was produced by transfection of Phoenix-ECO cells (ATCC CRL-3214) with Lipofectamine 2000 (ThermoFisher 11668019) according to manufacturer’s instructions. After 48 h, 1 ml of viral supernatant was used to infect primary myoblasts. After 48 h, infected myoblasts were selected with 3 µg.mL −1 of puromycin for 5 days and maintained on 0.5 µg.mL −1 of puromycin. For transient knockdown experiments, primary myoblasts were transfected twice with a 24-h interval, with 5 nM of a scrambled universal negative control siRNA or with 5 nM of siRNA targeting Mll1 , Mll2 , Set1a , or Set1b (Tri FECT a TM Dicer-Substrate RNAi kit, IDT), using Lipofectamine RNAiMax (Invitrogen). Transfected myoblasts were collected 24 h after the second transfection for RNA extraction. RT-qPCR and gene expression analysis For primary myoblasts, RNA was extracted using the Nucleospin RNA II kit (Macherey-Nagel), according to the manufacturer’s instructions. For satellite cells, RNA was isolated using Arcturus Picopure RNA extraction kit (Thermo Fisher Scientific). cDNA was synthesized using SuperScript III First-Strand Synthesis System (Invitrogen) by following the manufacturer’s protocol. Real-time quantitative PCR reactions were performed using iQ SYBR Green Supermix (Bio-Rad) and the CFX96 Real-Time PCR Detection System (Bio-Rad). A list of the primers used can be found in Supplementary Table 1 . For microarray analysis, RNA was purified as described above. Samples were hybridized to Affymetrix MoGene 1.0 ST chipsets (Affymetrix). Raw data were RMA normalized using the Bioconductor R package. The RMA normalized data was log2 transformed to determine fold change in gene expression. The following criteria were used to derive Table 1 : for downregulated genes, we chose genes exhibiting a log-fold change of greater than one (that is, twofold cut-off) and Affymetrix signal >7 for the higher signal; for upregulated genes, 10 most highly upregulated genes with Affymetrix signal >8 for the higher signal were selected; for myogenic genes, we selected genes with known roles in myogenesis with emphasis on homeodomain containing transcription factors, and not listed in other sections of table; for MLL1 target genes, Hox genes and few genes previously purported to be regulated by MLL1 were selected with Affymetrix signal >7. All Affymetrix probe set values are provided in Supplementary Data file 1 . Microarray data are available from the Gene Expression Omnibus, National Center for Biotechnology Information ( https://www.ncbi.nlm.nih.gov/geo/ ) under series GSE108339. Gene ontology analysis were performed using g:profiler ( https://biit.cs.ut.ee/gprofiler/gost ), and FIMO was employed to scan the Jaspar database for transcription factor binding sites within the Pax7 locus. Protein extraction and western blotting Primary myoblasts were lysed into RIPA buffer in the presence of EDTA-free Protease Inhibitor Cocktail (Roche). Histones were extracted from 2 × 10 6 primary myoblasts using the Histone Extraction Kit (ab113476, Abcam), according to the manufacturer’s instructions. Equal amounts of proteins or histone extracts were resolved on SDS-PAGE and transferred onto PVDF membranes. Membranes were blocked using 5% non-fat dry milk in TBS-Tween 0.1% for 1 h at room temperature followed by incubation with primary antibodies overnight at 4 °C. After four washes in TBS-Tween 0.1%, membranes were incubated 1 h with HRP-conjugated secondary antibodies. After four more washes, immunoblots were developed by enhanced chemiluminescence. A list of primary antibodies is available in Supplementary Table 3 . Full scans of the immunoblots are available in Supplementary Fig. 8 . Immunofluorescence Primary myoblasts and muscle cross-sections were fixed 5 min in 4% PFA solution in PBS, permeabilized in 0.1 M Glycine, 0.1% Triton X-100 in PBS for 10 min and blocked in either 5% horse serum, 2% BSA in PBS, or in 5% goat serum, 2% BSA, MOM blocking reagent 1:40, in PBS for 1 h at room temperature. 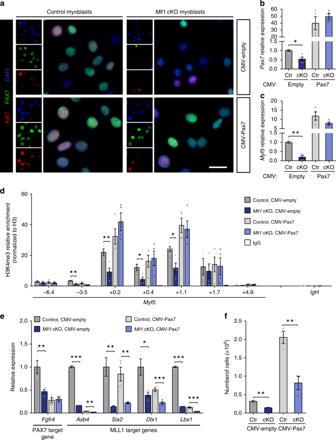Fig. 4 Overexpression of PAX7 restoresMyf5expression and H3K4me3 marks atMyf5locus inMll1cKO myoblasts.aImmunostaining of PAX7 (green) and Ki67 (red) in control andMll1cKO primary myoblasts transduced with either an empty plasmid or a CMV-Pax7 plasmid. Nuclei are counterstained with DAPI (blue). Scale bars represent 20 µm.b,cRT-qPCR analysis of (b)Pax7and (c)Myf5mRNA expression performed on control andMll1cKO primary myoblasts transduced with either an empty plasmid or a CMV-Pax7 plasmid, represented as mean ± S.E.M. (n= 4 independent experiments).dChIP-qPCR analysis of H3K4me3 enrichment, normalized to H3, atMyf5locus in control andMll1cKO primary myoblasts transduced with either an empty plasmid or a CMV-Pax7 plasmid. Values represent mean ± S.E.M. (n= 3 independent experiments).IgHenhancer region is used as a negative control.eRelative expression of PAX7 and MLL1 target genes in control andMll1cKO primary myoblasts transduced with either an empty plasmid or a CMV-Pax7 plasmid, represented as mean ± S.E.M. (n= 4 independent experiments).fNumber of control andMll1cKO primary myoblasts transduced with either an empty plasmid or a CMV-Pax7 plasmid. Cells were plated at the same density and grown for 6 days before enumeration. Values represent mean ± S.E.M. (n= 4 independent experiments) Primary antibodies were incubated overnight at 4 °C. After three washes in PBS, secondary antibodies were incubated in blocking buffer for 1 h at room temperature. Finally, muscle cross-sections were washed three times in PBS, nuclei were counterstained with DAPI (1:1000 in PBS), and slides were mounted with Permafluor. A list of primary and secondary antibodies is available in Supplementary Table 3 . Images of immunostaining were taken on a Zeiss Axio Observer.D1 inverted microscope equipped with either a Plan-Apochromat 20×/0.8 M27 objective or a Plan-Apochromat 63×/1.4.Oil DIC M27 objective. Images were processed and analyzed with Zen and FIJI software. Chromatin immunoprecipitation Primary myoblasts were cross-linked with 1% formaldehyde for 10 min at room temperature. Glycine was added to the fixing solution and incubated for 5 min. Cells were lysed in lysis buffer (50 mM Tris-HCl pH 8.0, 10 mM EDTA, 0.5% SDS) and chromatin was sheared using a Covaris sonicator. 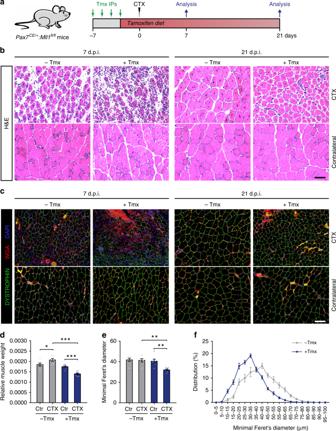Fig. 5 Genetic deletion ofMll1in satellite cells strongly impairs muscle regeneration.aExperimental schematic outlining the protocol followed to analyzed muscle regeneration ofPax7CE/+:Mll1fl/flmice.bHematoxylin and eosin (H&E) staining of cardiotoxin (CTX)-injured and contralateral (ctr)tibialis anterior(TA) muscles fromPax7CE/+:Mll1fl/flmice, treated or not with tamoxifen at 7 days or 21 days post-injury. Scale bar represents 100 µm.cWheat germ agglutinin (WGA, red) and DYSTROPHIN (green) staining of CTX-injured and contralateral TA muscles fromPax7CE/+:Mll1fl/flmice, treated or not with tamoxifen at 7 days or 21 days post-injury. Nuclei are stained with DAPI (blue). Scale bar represents 100 µm.dRelative CTX-injured and contralateral (ctr) TA muscle weight normalized to the body weight at 21 days post-injury, represented as means ± S.E.M (n= 7 mice per group).eMyofiber minimal Feret’s diameter of CTX-injured and contralateral (ctr) TA muscles fromPax7CE/+:Mll1fl/flmice treated or not with tamoxifen at 21 days post-injury, represented as mean ± S.E.M (n= 7 mice per group).fDistribution of minimal Feret’s diameter of CTX-injured TA muscles, as determined ine The sheared DNA was centrifuged at 13,000 × g for 5 min, and the remaining chromatin was diluted with an equal volume of dilution buffer (20 mM Tris-HCl pH 8.0, 1.2 mM EDTA, 1.1% Triton X-100, 200 mM NaCl). Chromatin was quantified using Bradford, and 500 µg of chromatin was used per chromatin immunoprecipitation (ChIP). Chromatin was pre-cleared for 30 min using protein A/G magnetic beads (30 µL per ChIP; Invitrogen). Antibodies (available in Supplementary Table 3 ) were added to the chromatin and incubated overnight with rotation at 4 °C. For transcription factor ChIP, 2 µg of anti-MLL1 N-terminal antibody or normal mouse IgG were used, and 2 µg of rabbit anti-mouse antibody was added to the reaction to amplify the signal. For histone modification ChIP, 5 µg of anti-Histone H3, anti-Histone H3K4me3 antibodies or normal rabbit IgG were used. The following day, protein A/G magnetic beads (30 µL per ChIP) were added to the lysate and incubated for 3 h with rotation at 4 °C. Beads were then washed three times with wash buffer (20 mM Tris-HCl pH 8.0, 150 mM NaCl, 2 mM EDTA, 0.1% SDS, 1% Triton X-100) for 5 min and two times with TE buffer for 5 min. DNA was eluted twice with freshly made elution buffer (0.1 M NaHCO 3 , 1% SDS) for 30 min. Eluates were pooled, and proteinase K was added to the chromatin and incubated overnight at 65 °C. DNA was purified by phenol/chloroform extraction. For ChIP in satellite cells, prospectively isolated satellite cells (CD31−, Cd11b−, SCA1−, CD45−, α7-Integrin+) were cross-linked and sonicated as described above. In total, 10 5 cells were used per ChIP, and 5% input was kept. Primary antibodies (2 µg of anti-H3K4me3 or rabbit IgG per ChIP) were pre-incubated with magnetic A/G beads (15 µL per ChIP) for 3 h with rotation at 4 °C. The antibody/bead complexes were incubated with chromatin for 2 h with rotation at 4 °C. 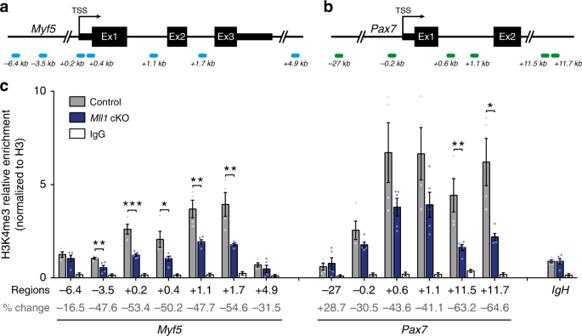Beads were washed as described above. Elution, reverse cross-link and proteinase K digestion were performed in a single step for 2 h at 65 °C, using Micro-ChIP Elution buffer (20 mM Tris-HCl pH7.5, 50 mM NaCl, 5 mM EDTA, 1% SDS, 50 µg.mL −1 proteinase K). 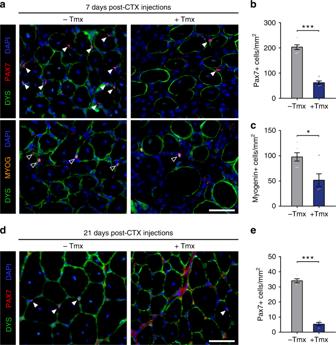Fig. 6 MLL1 is required for satellite cell proliferation and maintenance of the satellite cell pool.aImmunostaining with PAX7 (red) and MYOGENIN (orange) showing a markedly reduced numbers of satellite cells (white arrows) and differentiated cells (empty arrows) after satellite cell-specific deletion ofMll1induced by tamoxifen treatment. DYSTROPHIN staining (green) delineates the myofibers. Nuclei are counterstained with DAPI (blue). Scale bar represents 50 µm.bQuantification of Pax7-expressing cells per mm² from injured TA muscles of untreated (n= 6 mice) or tamoxifen-treated (n= 5 mice)Pax7CE/+:Mll1fl/flmice at 7 days post-injury.cQuantification of MYOGENIN-expressing cells per mm² from injured TA muscle sections of untreated (n= 6 mice) or tamoxifen-treated (n= 5 mice)Pax7CE/+:Mll1fl/flmice 7 days post-injury.dImmunostaining with PAX7 (red) confirming the decreased number of satellite cells (white arrows) after satellite cell-specific deletion ofMll1induced by tamoxifen treatment. DYSTROPHIN staining (green) delineates the myofibers. Nuclei are counterstained with DAPI (blue). Scale bar represents 50 µm.eQuantification of Pax7-expressing cells per mm² from injured TA muscle sections of untreated or tamoxifen-treatedPax7CE/+:Mll1fl/flmice 21 days post-injury (n= 4 mice per group) 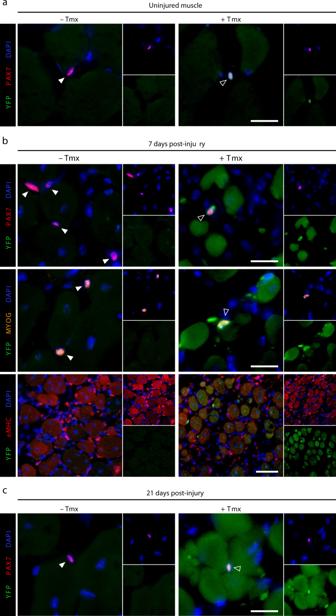Fig. 7 Mll1-deficient satellite cells retain their capacity to differentiate during muscle regeneration.aImmunostaining of PAX7 (red) showing satellite cells co-expressing YFP (green) upon 7-day tamoxifen treatment (+Tmx) in uninjured TA muscles fromPax7CE/+:Mll1fl/fl:RosaYFPmice. Untreated mice (− Tmx) do not exhibit any YFP staining. Nuclei are stained with DAPI (blue). Scale bar represents 20 µm.bTop and mid panel: satellite cells expressing either PAX7 (red) or MYOGENIN (orange), co-stained with YFP (green), of CTX-injured TA muscles fromPax7CE/+:Mll1fl/fl:RosaYFPmice treated or not with tamoxifen at 7 days post-injury. Nuclei are counterstained with DAPI (blue). Scale bar represents 20 µm. Lower panel: immunostaining of embryonic MHC (eMHC, red) for regenerating myofibers and YFP (green) at 7 days post-injury. Scale bar represents 50 µm.cPAX7 (red) and YFP (green) immunostaining of CTX-injured TA muscles fromPax7CE/+:Mll1fl/fl:RosaYFPmice treated or not with tamoxifen at 21 days post-injury. DAPI stained the nuclei (blue). Scale bar represents 20 µm. Throughout, white arrows and empty arrows indicate wild-type andMll1knockout satellite cells, respectively DNA was purified using the Nucleospin Gel and PCR Cleanup with NTB buffer (Macherey-Nagel). Fig. 2 Loss of MLL1 decreases H3K4me3 marks atMyf5andPax7loci inMll1cKO myoblasts.aLocation of primer sets relative toMyf5transcription start site (TSS) for ChIP-qPCR analysis ofMyf5promoter.bLocation of primer sets relative toPax7TSS and its downstream region for ChIP-qPCR analysis ofPax7promoter.cChIP-qPCR analysis of H3K4me3 enrichment, normalized to total H3, atMyf5andPax7loci in control andMll1cKO myoblasts, obtained after 4OHT-treated or EtOH-treatedRosaCE/+:Mll1fl/flmyoblasts (n= 5 independent experiments).IgHenhancer region is used as a negative control. Percent change in H3K4me3 enrichment between control andMll1cKO myoblasts is indicated for each region DNA enrichment was quantified by qPCR using the primers in Supplementary Table 2 . Statistical analysis Statistical evaluation was performed using the Student’s t -test tests to calculate differences between two groups and either one-way or two-way ANOVA with post hoc test for multiple comparisons (Graphpad Prism®). Data are presented as mean ± S.E.M. and p -value < 0.05 was considered as statistically significant. Throughout the paper, level of significance is indicated as follows: * p ≤ 0.05, ** p ≤ 0.01, *** p ≤ 0.001. Reporting summary Further information on research design is available in the Nature Research Reporting Summary linked to this article.